Vibrational nano-spectroscopic imaging correlating structure with intermolecular coupling and dynamics Molecular self-assembly, the function of biomembranes and the performance of organic solar cells rely on nanoscale molecular interactions. Understanding and control of such materials have been impeded by difficulties in imaging their properties with the desired nanometre spatial resolution, attomolar sensitivity and intermolecular spectroscopic specificity. Here we implement vibrational scattering-scanning near-field optical microscopy with high spectral precision to investigate the structure–function relationship in nano-phase separated block copolymers. A vibrational resonance is used as a sensitive reporter of the local chemical environment and we image, with few nanometre spatial resolution and 0.2 cm −1 spectral precision, solvatochromic Stark shifts and line broadening correlated with molecular-scale morphologies. We discriminate local variations in electric fields between nano-domains with quantitative agreement with dielectric continuum models. This ability to directly resolve nanoscale morphology and associated intermolecular interactions can form a basis for the systematic control of functionality in multicomponent soft matter systems. Many classes of soft matter gain their unique functionality from intrinsic or engineered inhomogeneities on nanometre-length scales. In particular, the phase behaviour of multicomponent nanoscale molecular composites such as biomembranes, organic photovoltaic systems, liquid crystals and polymer heterostructures are defined by intra- and intermolecular interactions. This intermolecular coupling dictates local morphology and vice versa. Precisely that complex microscopic interplay, in particular when associated with internal hetero-interfaces [1] , controls the macroscopic properties and performance of many materials. The general challenge and opportunity of controlling rich molecular-scale correlations in functional soft matter systems is exemplified in understanding the amphiphilic self-assembly of block copolymers (BCPs), which phase separate into a wide range of domain textures on macromolecular (3–150 nm)-length scales [2] . Many potential applications for photonic crystals, lithographic templates and engineered membranes are limited by nanoscale defects and disorder in the self-assembled morphologies of BCPs [3] . The phase separation of BCPs results in different local densities, degrees of crystallinity and chemical environments for specific functional groups between the centre and interface of a polymer block domain. Several established techniques such as grazing incidence X-ray diffraction, small/wide angle X-ray scattering [4] , near-edge X-ray absorption fine structure microscopy [5] , transmission electron microscopy, electron tomography and various scanning probe microscopies [6] give access to nanoscale morphology in soft matter. Despite these advances, simultaneous insight into the underlying spatial inhomogeneity of intermolecular coupling, charge transfer and their corresponding dynamics has remained difficult. In that regard, vibrational spectroscopies, such as vibrational Raman [7] and linear or multidimensional infrared [1] , are exquisitely sensitive to local chemical environments. However, these techniques in their conventional implementation do not provide nanoscale spatial information and only indirectly characterize the correlation of local morphology with molecular coupling [8] . Vibrational spectroscopic characterization is thus needed with chemical selectivity, high spectral precision, attomolar sensitivity and nanometre spatial resolution on the morphological length scales, which determine the function of soft-matter systems [9] , [10] , [11] , [12] . Here we perform nanometre-scale chemical imaging of domain morphology with simultaneous spectroscopic insight into underlying intermolecular coupling and associated dynamics. We achieve nanoscale chemical contrast through infrared vibrational scattering scanning near-field optical microscopy ( s -SNOM). Furthermore, using the high spectral power and resolution of a tunable quantum cascade laser, we extend infrared s -SNOM to true multispectral imaging (two spatial, one spectral dimension) in order to probe spectral variations as a function of spatial BCP morphology with 0.2-cm −1 spectral precision at ~10 nm spatial resolution. With this technique, we create spatiospectral maps using carbonyl resonances to locally probe the differences in intermolecular interactions at interfaces and within the nano-domains of quasi-lamellar poly(methyl methacrylate) (PMMA) in thin films of poly(styrene- block -methyl methacrylate) (PS- b -PMMA). From spatial maps of the spectral position and lineshape of the carbonyl mode, we gain insight into local chemical environments of subensembles within the phase-separated morphology. Furthermore, spectroscopic imaging within the amorphous PMMA domains enables the discrimination of effects due to electrochemical heterogeneity native to a non-crystalline polymer from effects due to mixing (such as Stark shifts or line narrowing) near PS:PMMA domain boundaries. 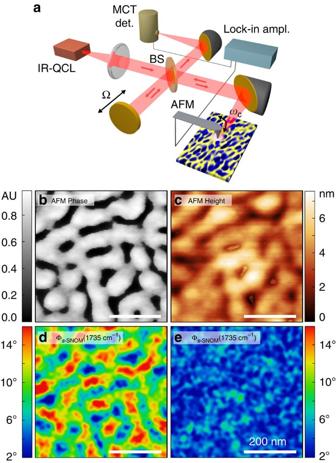Figure 1: Infrared vibrationals-SNOM imaging. (a) Diagram of interferometrics-SNOM experiment for spatiospectral nano-imaging, with atomic force microscope (AFM), tunable quantum cascade laser (QCL), MCT IR detector, beamsplitter (BS) and lock-in amplifier. Tip oscillation atωc~250 kHz, and reference arm mirror oscillation at Ω ~500 Hz. (b–e) Sample scans of quasi-lamellar PS-b-PMMA showing AFM tapping phase (b, arb. units), AFM height (c) and near-field phase (φs-SNOM) on (d) and off resonance (e) with the carbonyl mode (4-pixel Gaussian filter). Scale bars 200 nm. Experimental methods Figure 1a shows the layout of our experimental setup. Mid-infrared light from a quantum cascade laser (QCL, Daylight Solutions) tunable between 1,660 and 1,900 cm −1 with 0.2 cm −1 precision is focused on the apex of a Pt-coated tip (ARROW-NCPt, NanoWorld AG) of a modified atomic force microscope (AFM, Innova, Bruker) linearly polarized along surface normal relative to the sample, using an off-axis parabolic mirror (NA=0.4, effective focal length 19.5 mm), with a power density of ⩽ 50 MW cm −2 . Tip-scattered near-field signal is detected in a confocal epi-illumination/detection geometry with a HgCdTe detector (MCT, KLD-0.25/DC/11.5, Kolmar Technologies), and far-field background is suppressed by a lock-in filter (HF2, Zurich Instruments) demodulated at the third harmonic of the tip tapping frequency ω c . Tip-scattered light is recombined at the detector with light of known phase from the reference arm , in an asymmetric Michelson interferometer geometry. The near-field amplitude and phase are simultaneously determined by modulation of the reference phase at frequency Ω, similar to (ref. 13 ). and can then be related to the complex refractive index of the sample, as will be discussed below. For comparison, each sample was also measured using far-field ellipsometry, yielding ensemble-averaged spectra of the real and imaginary components of the complex index of refraction [14] . Figure 1: Infrared vibrational s -SNOM imaging. ( a ) Diagram of interferometric s -SNOM experiment for spatiospectral nano-imaging, with atomic force microscope (AFM), tunable quantum cascade laser (QCL), MCT IR detector, beamsplitter (BS) and lock-in amplifier. Tip oscillation at ω c ~250 kHz, and reference arm mirror oscillation at Ω ~500 Hz. ( b – e ) Sample scans of quasi-lamellar PS- b -PMMA showing AFM tapping phase ( b , arb. units), AFM height ( c ) and near-field phase ( φ s -SNOM ) on ( d ) and off resonance ( e ) with the carbonyl mode (4-pixel Gaussian filter). Scale bars 200 nm. Full size image A high molecular weight BCP of PS- b -PMMA with a relative chain length of 270.0- b -289.0 M n × 10 3 (P4443-SMMA, Polymer Source) is spin-coated from a 1% w/v solution in toluene on native-oxide silicon substrates (1–4 kRPM). Long chain lengths result in non-equilibrium, irregularly shaped quasi-lamellar domains with incomplete phase separation and large interfacial mixing regions [15] , [16] . Infrared vibrational contrast As shown in the AFM images ( Fig. 1b,c ), differences in the viscoelastic properties between PMMA and PS result in contrast between nanodomains of the two polymers, in tapping phase and topography [17] . Fig. 1d,e show simultaneously recorded near-field images of the s -SNOM phase with photon energy resonant (d) and non-resonant (e) with the carbonyl vibrational mode of PMMA. The strength of the s -SNOM phase signal is proportional to the resonant response of the sample, and can thus be used to map the local concentration of carbonyl groups. As the carbonyl resonance is found in PMMA and not PS ( Fig. 2b ), the s -SNOM phase is linearly related to the relative density of PMMA:PS within the ~10 3 nm 3 near-field probe volume of the tip [18] . This approximation is general for isotropically oriented molecules as in the case of the highly amorphous PS- b -PMMA copolymer. 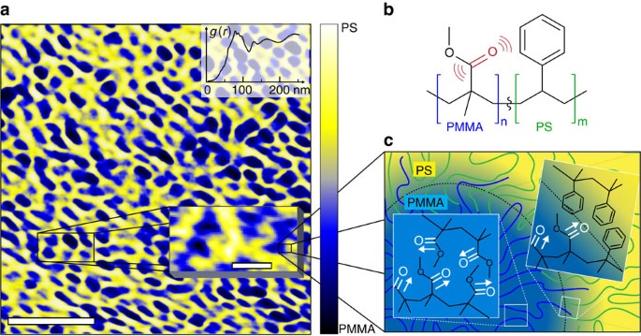Figure 2:s-SNOM image of nanoscale chemical morphology of block copolymer. (a) Nanoscale chemical map of self-phase separated amphiphilic block copolymer PS-b-PMMA derived from carbonyl resonants-SNOM imaging. Scale bar 750 nm. The radial distribution functiong(r) is obtained from the large area scan (top right inset). A high spatial resolution (scale bar 100 nm)s-SNOM image showing additional features and continuous variation in relative PMMA:PS density across the interface is overlaid. (b) Molecular structure of (PS-b-PMMA), highlighting the carbonyl marker resonance. (c) Schematic of domain morphology of PS-b-PMMA with incomplete segregation near the interface. Figure 2a illustrates the chemical contrast observed in a large area s -SNOM scan of PS-b-PMMA. Spatial Fourier analysis reveals a radial distribution function g ( r ) with a peak at 80±20 nm ( Fig. 2a , top inset), indicative of the length scale of microphase separation. A high spatial resolution image ( Fig. 2a , bottom inset) shows additional morphological details within the ~10-nm resolution limit. The relative density of PMMA in the high-resolution image is observed to vary across the nanodomain interface, over a typical length scale of 30–40 nm, as a result of the incomplete phase separation. As schematically shown in Fig. 2c , the associated spatial variation in local chemical environment is expected to give rise to observable changes in the spectroscopic signatures of the carbonyl oscillator as a reporter mode, between the centre and interfacial region of the domains. Figure 2: s -SNOM image of nanoscale chemical morphology of block copolymer. ( a ) Nanoscale chemical map of self-phase separated amphiphilic block copolymer PS- b -PMMA derived from carbonyl resonant s -SNOM imaging. Scale bar 750 nm. The radial distribution function g ( r ) is obtained from the large area scan (top right inset). A high spatial resolution (scale bar 100 nm) s -SNOM image showing additional features and continuous variation in relative PMMA:PS density across the interface is overlaid. ( b ) Molecular structure of (PS- b -PMMA), highlighting the carbonyl marker resonance. ( c ) Schematic of domain morphology of PS- b -PMMA with incomplete segregation near the interface. Full size image Multispectral imaging Multispectral s -SNOM optical phase images of a 500 nm × 225 nm region of a quasi-lamellar PS- b -PMMA film are obtained by sequential sample scanning ( Fig. 3a ) and tuning across the carbonyl resonance from 1,660 to 1,800 cm −1 in 3 cm −1 increments. The characteristic carbonyl resonance gives rise to a continuous variation of s -SNOM spectral phase and amplitude when self-referenced to non-resonant PS (which exhibits a low and flat response in this spectral range). 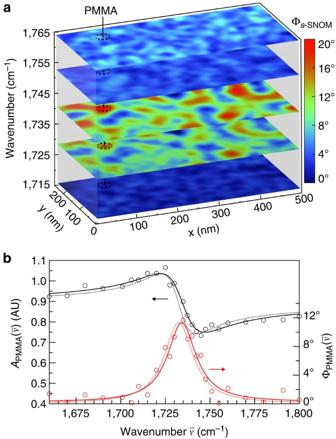Figure 3: Spatiospectral nano-imaging. (a) Multispectrals-SNOM phase image of PS-b-PMMA. Carbonyl resonant PMMA region highlighted for illustration. Colour bar indicates spectral phase. (b)s-SNOM amplitudeand phasespectrum of a ~25 × 25 nm2PMMA region (referenced to a non-resonant PS region of similar size), with real and imaginary Lorentzian fits for the amplitude and phase, respectively (solid lines). Dotted lines show(black) and(red) from far-field spectroscopic ellipsometry, scaled vertically for comparison. Figure 3b shows the resulting s -SNOM spectrum of the nanoscale PMMA region indicated in (a). From the molecular density of PMMA of 6.2 monomer nm −3 and a near-field signal depth of ⩽ 10 nm corresponding to first order to the lateral spatial resolution [19] , [20] , this spectrum corresponds to a sub-ensemble of only 25 zeptomole of ~10 4 carbonyl oscillators. Figure 3: Spatiospectral nano-imaging. ( a ) Multispectral s -SNOM phase image of PS- b -PMMA. Carbonyl resonant PMMA region highlighted for illustration. Colour bar indicates spectral phase . ( b ) s -SNOM amplitude and phase spectrum of a ~25 × 25 nm 2 PMMA region (referenced to a non-resonant PS region of similar size), with real and imaginary Lorentzian fits for the amplitude and phase, respectively (solid lines). Dotted lines show (black) and (red) from far-field spectroscopic ellipsometry, scaled vertically for comparison. Full size image The peak centre of is slightly blue-shifted compared with the far-field ensemble spectrum of obtained from ellipsometry due to the spectral phase approximation [21] , [22] . The shift amounts to only a few wavenumbers in PMMA because the large off-resonant contributions to the dielectric function in the infrared spectral range give rise to a comparably weak resonant dispersion. The near-field spectral phase is therefore approximately equal to the imaginary amplitude [22] , which is, in turn, proportional to the imaginary part of the sample dielectric function. This results in , to a good approximation [21] , [23] . Spatio-spectral image analysis The analysis of the nanoscale phase spectra in terms of resonance frequency and line width gives access to nanoscale variations in local chemical environment. 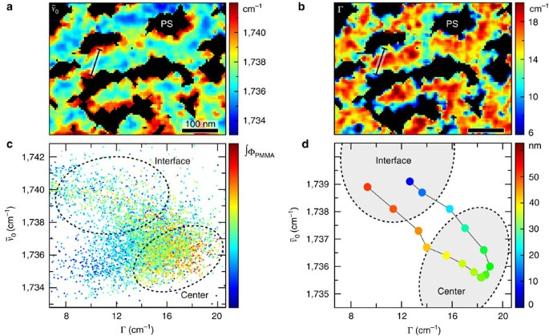Figure 4: Spatiospectral image analysis. (a,b) Image of carbonyl resonance frequency(a) and linewidth Γ (b). Black areas correspond to PS domains with too low PMMA density to be analysed. Scale bars 100 nm. (c) Scatterplot ofversus Γ of the data from (a,b), with colour code referring to spectral intensity integrated over the area of the peak in phase, corresponding to the oscillator density of PMMA. (d) Plot ofversus Γ for individual points along the 60-nm spatial profile indicated by the black line in (a,b), exemplifying the overall trend shown in (c), and illustrating the morphological trend underlying the observed spectral variation. Figure 4 shows the result of Lorentzian line fits from the complete multispectral scan of Fig. 3a , with extracted peak position (a) and full-width at half-maximum linewidth Γ (b) for each 10 nm × 10 nm pixel area. In general, a spectral red shift and broader linewidth is found towards the centre of PMMA domains, compared with a blue-shifted and narrower spectral response at domain interfaces. Figure 4: Spatiospectral image analysis. ( a , b ) Image of carbonyl resonance frequency ( a ) and linewidth Γ ( b ). Black areas correspond to PS domains with too low PMMA density to be analysed. Scale bars 100 nm. ( c ) Scatterplot of versus Γ of the data from ( a , b ), with colour code referring to spectral intensity integrated over the area of the peak in phase, corresponding to the oscillator density of PMMA. ( d ) Plot of versus Γ for individual points along the 60-nm spatial profile indicated by the black line in ( a , b ), exemplifying the overall trend shown in ( c ), and illustrating the morphological trend underlying the observed spectral variation. Full size image Despite some spatial inhomogeneities in the degree of resonance shifts and line broadening, a clear difference between spectra within domain centres compared with interfacial regions is evident when considering the ensemble distribution of pixels over the entire spatiospectral image. As shown in Fig. 4c , a correlation plot of versus Γ separates points of varying carbonyl oscillator density with associated spatial regions by the integrated spectral phase (colour bar). It shows the trend of redshifting and broadening towards the domain centres, which are characterized by higher carbonyl oscillator density. As a specific example, Fig. 4d shows the distinct centre versus interfacial behaviour across a single domain covering a 60-nm distance as indicated in Fig. 4a,b (black line). The peak is observed to monotonically redshift and broaden towards the centre of the domain, and blueshift and narrow towards the interface. Note that this effect is opposite to a spectral shift associated with the spectral phase approximation where the s -SNOM peak position would either be unchanged or red-shifted towards the actual resonance frequency, depending on the effect of dilution of carbonyl oscillators in the PMMA/PS mixture on the non-resonant contribution to the dispersion . Nanoscale-resolved solvatochromism We attribute the red shift towards the centre of PMMA domains to a spatially varying Stark shift, caused by heterogeneity in the local chemical environment. Stark effect-induced red shift of the carbonyl mode is proportional to the local electric field ‹ F › given by: A change in dipole moment upon photoexciation, Δ μ probe , also termed the Stark tuning rate, results in a red shift of the reporter mode with increasing field strength [24] . Carbonyl modes have a large Stark tuning rate, and thus enable the methyl-ester group of the PMMA polymer to act as a particularly sensitive reporter of local electric field strength. Thus, the observed red shift of the carbonyl vibration towards the centre of the PMMA domains indicates larger local electric fields within the domains relative to their interface. Solvation and solvatochromism of polar molecules can be described by dielectric continuum models, which have successfully been applied to quantitatively describe, for example, local structure and intramolecular electric fields in proteins [24] . In the Onsager model of solvation, which describes electric fields within the solvation shell surrounding a polar solute molecule, the local electric field F surrounding a dipolar solute is proportional to the dipole moment of the molecule μ , modified by its refractive index n , and the dielectric constant ε of the solvent [25] , and given by where a is the solvation shell radius of the solute molecule and can be approximated from bulk densities. Within this model, we can describe the solute probe as a segment of a syndiotactic PMMA chain with a dipole moment oriented along the carbonyl bond of the methacrylate group ( Fig. 2c white arrows). Solvatochromism of its carbonyl group results from changes in the local dielectric environment due to mutual self-interaction of neighbouring methyl-ester groups of PMMA. Owing to the large chain length in our high molecular weight BCP, incomplete phase separation and significant mixing occurs near the interface, and the local dielectric constant is a continuously varying function of PS:PMMA ratio across the interface region. The dielectric constant of PS is lower than that of PMMA, and thus red shifts are expected with increasing local density of PMMA relative to PS. Local chemical environment As seen from the correlation plot in Fig. 4 (c), the carbonyl mode redshifts by ~3 cm −1 measured in the PMMA-dense domain centres, relative to the PS-rich inferface regions. Using literature values for the dielectric properties of PMMA and PS, we compare our results to predictions from the Onsager model. Spectral shifts measured with s -SNOM are aligned with Onsager fields calculated using bulk dielectric parameters of s -PMMA and PS. 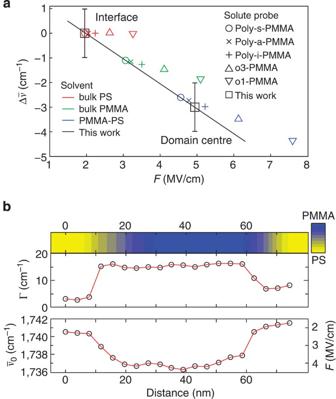Figure 5: Intermolecular field and nanoscale variation of coupling and dynamics. (a) Modelled solvatochromic spectral shifts of the carbonyl resonance relative to the shift predicted for a molecular probe in bulk PS. Electric field and Stark shift are calculated for dielectric environments in PS (red), bulk PMMA (green)36and PMMA nano-domains in a PS-PMMA blend (blue)29. The molecular probe is approximated using dielectric parameters for various tacticities of PMMA, syndiotactic- (circle), atactic- (x) or isotactic- (+) PMMA chains, as well as for shorter oligomer segments (trimer o3-PMMA) and monomer (o1-PMMA). Locals-SNOM measurement of spectral shift in domain centres relative to the interface for syndiotactic-PS-b-PMMA are indicated by black squares, with error bars calculated from the spectral distribution of peak positions in centre and interface. (b) Spectrally resolved line cut along the region indicated inFig. 4a,bshowing local relative concentration of PMMA as measured by thes-SNOM phase (top colour map), linewidth (middle), and spectral shift (bottom), with derived local electric fieldF. Figure 5a shows that the local electric field surrounding the carbonyl group is expected to increase from ~2 MV cm −1 in PS to ~5 MV cm −1 in PMMA. On the basis of these modelled local electric field strengths between centre and interface, and the range of observed shifts in Fig. 4 (c), we derive, using equation 2, a Stark tuning rate of Δ μ ~1 cm −1 /(MV/cm). This value is consistent with literature values [26] , [27] . Figure 5: Intermolecular field and nanoscale variation of coupling and dynamics. ( a ) Modelled solvatochromic spectral shifts of the carbonyl resonance relative to the shift predicted for a molecular probe in bulk PS. Electric field and Stark shift are calculated for dielectric environments in PS (red), bulk PMMA (green) [36] and PMMA nano-domains in a PS-PMMA blend (blue) [29] . The molecular probe is approximated using dielectric parameters for various tacticities of PMMA, syndiotactic- (circle), atactic- (x) or isotactic- (+) PMMA chains, as well as for shorter oligomer segments (trimer o3-PMMA) and monomer (o1-PMMA). Local s -SNOM measurement of spectral shift in domain centres relative to the interface for syndiotactic-PS- b -PMMA are indicated by black squares, with error bars calculated from the spectral distribution of peak positions in centre and interface. ( b ) Spectrally resolved line cut along the region indicated in Fig. 4 a , b showing local relative concentration of PMMA as measured by the s -SNOM phase (top colour map), linewidth (middle), and spectral shift (bottom), with derived local electric field F . Full size image The microscopic spatial variations of the experimentally measured Stark shift span a broad distribution, yet a comparable distribution of local electric field strengths can be predicted through the Onsager model, as shown in Fig. 5a . This distribution occurs because bulk properties of a polymer depend heavily on structural details of the polymer chain rather than simply on the monomeric chemical identity. Different stereocomplexes of PMMA, isotactic ( i -PMMA), atactic ( a -PMMA), and syndiotactic ( s -PMMA) that are used here differ only in chirality, yet i -PMMA has a larger mean-square dipole moment ‹ μ 2 › due to a larger degree of chain order. Measured bulk values of ‹ μ 2 › are also heavily dependent upon chain length; monomers (o1-PMMA) or oligomers (trimeric o3-PMMA) of PMMA have larger ‹ μ 2 › and thus are expected to undergo larger Stark shift in the same local solvent environment as compared with longer chains [28] . Morphologically induced ordering also affects dielectric properties, and PMMA nanodomains in PS-PMMA copolymers have been observed to have unusually large dielectric permittivity as evidenced by large Stark shifts of a dye molecule probe [29] . Rotation of individual monomers, local fluctuations in density [9] , and increased chain mobility within 10–50 nm of a surface also affect the dielectric properties [11] , [12] . Variation in local chemical environment is thus expected for nanoscale subensembles of a polymer blend with molecular scale disorder. The continuum description thus acts as a lower bound for predicted spectral shifts. The spectral shifts observed in s -SNOM thus quantitatively agree with the model of solvation-induced DC Stark shift. Indeed, nanoscale inhomogeneities in measured spectral shifts and linewidths can be expected and fall within shifts expected from variation of bulk dielectric properties of PMMA. Further microscopic insight can be obtained from mapping changes in density and changes in line shape across a single domain. The PMMA local density ( Fig. 5b top, as obtained from the resonant s -SNOM phase) is measured simultaneously with the linewidth ( Fig. 5b , middle) and peak centre of the carbonyl stretch ( Fig. 5b , bottom). Using the value for the Stark tuning rate of Δ μ =cm −1 (MV/cm), shifts in the peak centre can be associated with reaction field strength ( Fig. 5b bottom, right scale). Although other significant factors and structural details contribute significantly as discussed above, the peak shift correlates with mixing ratio across the image or within a single line cut as modelled by a Stark shift. Heterogeneity-induced Stark shifts have been recently observed in a number of polymer and thin film systems with far-field spectroscopies [30] . In particular, time-resolved infrared spectroscopy in poly-3-hexyl-thiophene: phenyl-C61-butyric acid methyl ester (P3HT:PCBM) bulk heterojunctions [26] , found a dynamic red shift in the methyl ester stretch of PCBM following charge separation, which was attributed to higher field strengths in PCBM domain centres compared with interfaces. Conversely, annealing-induced changes in morphology of a P3HT: PCBM resulted in Stark shifts of the methyl-ester stretch as observed via linear far-field infrared spectroscopy, which was attributed to increased electric field strengths at the interface (rather than domain centre) as a result of increased conductivity and decreased screening lengths [27] . With our spatiospectral implementation of infrared s -SNOM, we overcome difficulties in assigning mophologically induced spectral features. We are able to image and thus directly correlate morphology and spectral signatures, conclusively assigning red shifts and broadening to changes in local chemical environment at domain centres. In addition to spectral red shifts, we find a correlation between vibrational linewidth and position relative to domain boundaries, with line broadening in the domain centre, as seen in the correlation plot ( Fig. 4c,d ) and line cut ( Fig. 5b ). We believe that this is a result of both increased and inhomogeneous solute-bath coupling, and the availability of additional nearly degenerate and low-energy modes that contribute to faster vibrational dephasing (when compared with the domain interface with its generally low density and thus weakly coupled carbonyl resonances). Strength of solvation is commonly correlated with both red shift of the solute mode and spectral broadening as a result of increased system-bath coupling [31] . Competing and opposing contributions to linewidth, however, can complicate such a simple picture. Contributions to homogeneous and inhomogeneous broadening result from varying molecular order and a complex interplay of attractive and repulsive intermolecular forces [32] , coupling of the vibrational mode and molecular dipole moment to the bath as a function of density [33] , and temperature effects in activated vibrational energy transfer [34] . Inverse correlation between solvent polarity and spectral linewidth has been observed with far-field infrared spectroscopy in cases where increases in vibrational linewidths due to vibrational dephasing are overwhelmed by narrowing of slower dynamical process involved in spectral diffusion [35] . In PS- b -PMMA, our results suggest that increased intra- and interchain coupling within the PMMA domains seems to increase both vibrational linewidth and Stark shift relative to the PS-rich interfacial regions. In summary, we have implemented multispectral infrared-vibrational near-field imaging as a nano-chemometric tool to spatially resolve intermolecular interaction with nanometre spatial resolution, attomolar sensitivity and sub-wavenumber spectral precision. The approach is on the basis of vibrational linewidth, lifetime and resonant frequency, being exquisitely sensitive to intra- and intermolecular interactions, opening direct spectroscopic access to nanoscale bulk and nanointerfaces in heterogeneous multicomponent soft matter. It thus provides direct molecular level insight into the elementary processes linking morphology with intra- and intermolecular coupling and resulting macroscopic material properties. Infrared-vibrational nano-chemometrics with full spatiospectral analysis and its possible extension to ultrafast, time-domain implementations can thus provide deep insight into degrees of disorder, crystallinity, strain, stoichiometry, charge transfer, solvatochromism and other processes that underlie the structure–function relationship of essentially all soft-matter systems. How to cite this article: Pollard, B. et al . Vibrational nano-spectroscopic imaging correlating structure with intermolecular coupling and dynamics. Nat. Commun. 5:3587 doi: 10.1038/ncomms4587 (2014).